Strengthening effect of single-atomic-layer graphene in metal–graphene nanolayered composites Graphene is a single-atomic-layer material with excellent mechanical properties and has the potential to enhance the strength of composites. Its two-dimensional geometry, high intrinsic strength and modulus can effectively constrain dislocation motion, resulting in the significant strengthening of metals. Here we demonstrate a new material design in the form of a nanolayered composite consisting of alternating layers of metal (copper or nickel) and monolayer graphene that has ultra-high strengths of 1.5 and 4.0 GPa for copper–graphene with 70-nm repeat layer spacing and nickel–graphene with 100-nm repeat layer spacing, respectively. The ultra-high strengths of these metal–graphene nanolayered structures indicate the effectiveness of graphene in blocking dislocation propagation across the metal–graphene interface. Ex situ and in situ transmission electron microscopy compression tests and molecular dynamics simulations confirm a build-up of dislocations at the graphene interface. Enhancing the strength of metals through microstructure engineering is of critical importance for the development of structural materials. The key factor that determines the strength of the metal is how effectively dislocation motion can be hindered; the well-known Hall–Petch relationship describes how polycrystalline metals become stronger as grain size is reduced [1] , [2] . Recently, researchers have studied metal nanolayered composite systems, the strength of which can be enhanced by introducing a high density of interfaces that block dislocation motion [3] , [4] , [5] , [6] , [7] , [8] . A metal nanolayered composite with discontinuous crystallographic planes, known as an incoherent interface system (for example, [111]Cu–[110]Nb), provides increased resistance against dislocation propagation across the interface [8] , [9] , [10] . In addition, atomistic studies of incoherent multilayers have reported a ‘self-healing’ ability that annihilates dislocations at the interfaces through core dissociation processes. This ‘self-healing’ mechanism has been proposed to depend on the interfacial strengths [9] , [10] . Carefully engineered nanolayered composites have various applications; the nuclear reactor structural material application is especially promising due to the high strength and ‘self-healing’ ability of the nanolayered composites [8] , [9] , [10] . Graphene is a single-atomic-layer material with excellent mechanical properties, with the highest-known intrinsic strength of 130 GPa and a Young’s modulus of 1 TPa [11] , [12] , [13] , [14] . It also has well-known electrical properties, including a mobility of ~15,000 cm 2 V −1 S −1 and a non-doped sheet resistance of ~350 Ohm per square [12] , [13] , [14] , [15] , [16] . Graphene has excellent potential as a strength enhancer in composites owing to its two-dimensional (2D) geometry and high mechanical strength and modulus. Most of the previous research has been focused on synthesizing simple mixtures of graphene flakes that are reduced from graphene oxide in a polymer [17] , [18] or metal [19] matrix. However, the low mechanical strength of graphene oxide [20] and the insufficient, non-uniform dispersion of graphene flakes within the matrix result in relatively poor strength enhancement [19] . If one assumes a simple rule of mixture, where , the resulting strength enhancement of a randomly distributed graphene composite is expected to be small for 0.1–1.0 wt% graphene [18] . However, if the graphene can be incorporated into a metal–graphene layered composite system, then the strengthening effect can reach far beyond the simple rule of mixture, as has been evidenced by previous reports on metal nanolayered systems [3] that reported a high degree of strengthening by reducing the layer spacing while maintaining the volume fraction of the layers. In this study, we report for the first time the development of a metal–graphene nanolayered composite that utilizes the key advantages of graphene, including ultra-high strength, modulus and 2D geometry, as a strength enhancer. The mechanical properties of the synthesized metal–graphene nanolayered composites are measured using nanopillar compression testing [21] , and subsequent transmission electron microscopy (TEM) analysis and in situ TEM compression testing provide insight into the deformation mechanisms. To further understand the interaction of the dislocations at the metal–graphene interfaces, molecular dynamics (MD) simulations were performed to gain a fundamental understanding of the role of graphene during deformation. We clearly demonstrate that our new metal–graphene nanolayered composite showed ultra-high strength because the graphene provides an efficient barrier to dislocation motion across the interface. Synthesis of metal–graphene nanolayered composites A previously reported chemical vapour deposition (CVD) method was used to grow the graphene layers [22] for the metal–graphene nanolayered composites. Raman spectroscopy ( Supplementary Fig. S1 ) confirmed that the resulting graphene was mostly a single (85%) atomic layer with a reasonable G/2D ratio of 1/2.15. Next, the graphene was transferred to a metal-deposited substrate via a PMMA support layer, which was subsequently removed after the transfer. By repeating the above steps, we synthesized Cu–graphene nanolayered composites with varying repeat layer spacings of 70, 125 and 200 nm and Ni–graphene nanolayered composites with repeat layer spacings of 100, 150 and 300 nm ( Fig. 1 ). Detailed cross-sectional TEM images and histograms of line scans across the interface using a high-voltage electron microscope (HVEM) are shown in Fig. 2a ; the images indicate the presence of both single (region (A)) and double (region (B)) layers of graphene. Only a single high-intensity peak was observed in region (A), whereas two high-intensity peaks separated by the expected interplanar spacing of 0.34 nm were observed in region (B). These results agree with the Raman results in Supplementary Figure S1 . 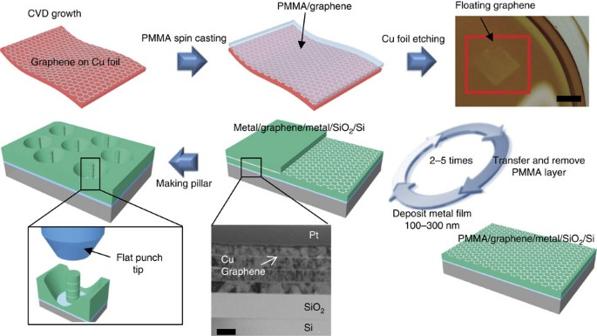Figure 1: Schematic of metal–graphene multilayer system synthesis. Graphene is first grown using CVD and transferred onto the evaporated metal thin film on an oxidized Si substrate. The PMMA layer is then removed, and the next metal thin film layer is evaporated. By repeating the metal deposition and graphene transfer processes, Cu–graphene nanolayered composites are synthesized with different repeated metal thicknesses of 70, 125 and 200 nm, and Ni–graphene nanolayered composites are synthesized with repeated metal thicknesses of 100, 150 and 300 nm. The mechanical properties were studied by compression testing of nanopillars etched by FIB. The scale bar for the floating graphene is 10 mm and that for the TEM is 200 nm. Figure 1: Schematic of metal–graphene multilayer system synthesis. Graphene is first grown using CVD and transferred onto the evaporated metal thin film on an oxidized Si substrate. The PMMA layer is then removed, and the next metal thin film layer is evaporated. By repeating the metal deposition and graphene transfer processes, Cu–graphene nanolayered composites are synthesized with different repeated metal thicknesses of 70, 125 and 200 nm, and Ni–graphene nanolayered composites are synthesized with repeated metal thicknesses of 100, 150 and 300 nm. The mechanical properties were studied by compression testing of nanopillars etched by FIB. The scale bar for the floating graphene is 10 mm and that for the TEM is 200 nm. 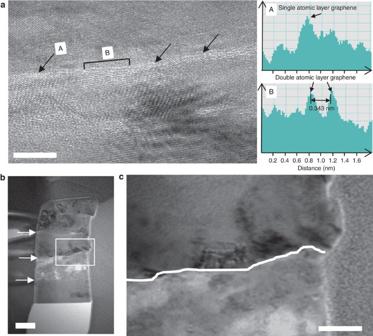Figure 2: TEM analysis of the Cu–graphene nanolayered composite. (a) TEM image of a metal–graphene interface that shows mostly single layers with some double layers. Scale bar, 5 nm. (b) TEM image of a Cu–graphene nanopillar with 125-nm repeat layer spacing at a low magnification after deformation. Scale bar, 100 nm. (c) TEM image of a Cu–graphene nanopillar after deformation that shows a higher density of dislocations above the graphene interface. Scale bar, 50 nm. Full size image Figure 2: TEM analysis of the Cu–graphene nanolayered composite. ( a ) TEM image of a metal–graphene interface that shows mostly single layers with some double layers. Scale bar, 5 nm. ( b ) TEM image of a Cu–graphene nanopillar with 125-nm repeat layer spacing at a low magnification after deformation. Scale bar, 100 nm. ( c ) TEM image of a Cu–graphene nanopillar after deformation that shows a higher density of dislocations above the graphene interface. Scale bar, 50 nm. Full size image Ultra-high strength shown by nanopillar compression To test the mechanical properties of the metal–graphene nanolayered composites, nanopillar compression tests developed by Uchic et al . [21] were performed. Focused ion beam (FIB) milling was utilized to fabricate nanopillars with a diameter of 200 nm and height of 400–600 nm. Scanning electron microscope images of a Cu–graphene nanopillar with 125-nm repeat layer spacing before and after compression testing are shown in Fig. 3a . Here, the nanopillar compression test is used to evaluate the mechanical behaviour of the nanolayered composites in the absence of any strain gradient effects. We control for the FIB modification of material properties and the well-documented size-dependent plasticity of single-crystal metal nanopillars [21] , [23] , [24] by milling all nanopillars to the same diameter, which was chosen to be larger than the repeat layer spacings of the nanolayers. In addition, the grain size analysis of the Cu–graphene samples indicated that the average grain sizes ranged from 143 to 125 nm for repeat layer spacings from 194 to 200 nm ( Supplementary Fig. S2 ). Therefore, each 200-nm-diameter nanopillar is expected to be composed predominantly of a single grain or double grains at most. The single-grain nature of the nanopillars can also be observed in the TEM micrograph of the Cu–graphene nanopillar shown in Supplementary Figure S3 . Thus, the only systematically varying length scale for plastic deformation is the interlayer spacing of the nanolayered composites. 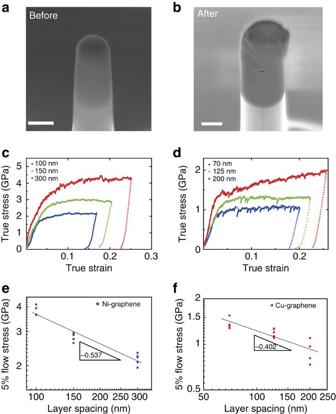Figure 3: Results of nanopillar compression test. Scanning electron microscope image of a Cu–graphene nanopillar with 125-nm layer spacing (a) before and (b) after compression testing. Scale bar, 200 nm. Stress versus strain curves for (c) Ni–graphene and (d) Cu–graphene of various repeat metal layer spacings. The flow stresses at 5% plastic strain versus repeat layer spacing plots for (e) Ni–graphene and (f) Cu–graphene nanolayered composites. Figure 3: Results of nanopillar compression test. Scanning electron microscope image of a Cu–graphene nanopillar with 125-nm layer spacing ( a ) before and ( b ) after compression testing. Scale bar, 200 nm. Stress versus strain curves for ( c ) Ni–graphene and ( d ) Cu–graphene of various repeat metal layer spacings. The flow stresses at 5% plastic strain versus repeat layer spacing plots for ( e ) Ni–graphene and ( f ) Cu–graphene nanolayered composites. Full size image The results of the nanopillar compression tests of the Cu– and Ni–graphene composites are shown in Fig. 3c . The stress versus strain response was evaluated using a constant-volume, homogeneous deformation model [23] . It is striking to note that the strengths of both the Ni– and Cu–graphene nanolayered composites are extremely high and that the flow stresses systematically increase with a reduction in metal layer spacing. The highest strengths were observed for the smallest metal layer spacing; the Cu– and Ni–graphene nanopillars exhibited an average flow stress at 5% plastic strain of 1.5 and 4.0 GPa, respectively. These values are in excess of a few hundred times the yield strength of the respective bulk single-crystal metals. For the 100-nm Ni–graphene nanolayered composites, the flow stresses at 5% plastic strain were as high as 52% of the theoretical shear strength [25] of Ni as given by G /10=7.6 GPa, where G is the shear modulus. The flow stresses at 5% plastic strain were extracted for the Cu– and Ni– graphene nanopillars and plotted against the corresponding metal layer spacing in Fig. 3e ; there is a clear trend in strength enhancement with a reduction in metal repeat layer spacing. The slopes of the log–log plot of 5% flow stress versus strain for the Cu– and Ni–graphene are −0.402 and −0.537, respectively, and are in close agreement with the Hall–Petch [26] exponent, , where h is the repeat layer thickness. This finding suggests that multiple dislocations pile up at the interface, consistent with previous studies on metal nanolayered composites that demonstrated a Hall–Petch-like behaviour at a length scale greater than 100 nm (refs 4 , 5 , 26 ). In the conventional sense of the Hall–Petch strengthening mechanism, dislocations pile up at the interface and eventually propagate through the interface when a critical shear stress is applied. The critical event in the case of our metal–graphene nanolayered composite would be the activation of complex slip systems at high stresses and/or the piled-up dislocations escaping through the free surface due to interfacial shear because of the extreme difficulty in shearing through the graphene layer, which is explained in more detail later in this manuscript. The deformed Cu–graphene nanopillars were further analysed using an HVEM to gain insight into the deformation mechanism that is responsible for the observed high strengths and strain-hardening behaviour. A bright-field TEM image of a Cu–graphene multilayer nanopillar after a compressive strain of 23% is shown in Fig. 2b ; the magnification of the highlighted area in the rectangle is shown in Fig. 2c . The interface between the Cu–graphene nanopillars after compression ( Fig. 2c ) indicates that a higher density of dislocations was present in the upper layer because the Cu–graphene interface acted as an effective barrier to dislocation propagation across the interface. In addition, we confirmed that the graphene was not sheared during deformation up to a total compressive strain of 23%. The high intrinsic mechanical strength of graphene prevented rupture and shearing; therefore, the graphene served as an efficient constraint to dislocation propagation across the interface. To further demonstrate the ability of a single atomic layer of graphene to efficiently block gliding dislocations, an in situ TEM nanopillar compression test was performed using a Hysitron Picoindenter (PI-95) in an FEI Tecnai G2 F20 microscope. The specimen used for the in situ TEM study contained one layer of graphene between two layers of Cu as shown in Fig. 4a . The compression was performed under displacement control with a nominal engineering strain rate of 0.002 (s −1 ). The in situ TEM movie in Supplementary Movie 1 and the TEM micrographs of the nanopillar before and after deformation shown in Fig. 4 clearly demonstrate that gliding dislocations were unable to penetrate the graphene interface. The in situ TEM compression movie in Supplementary Movie 1 shows that the lower Cu layer, which was 960 nm thick, showed dislocation starvation [23] , which was expected because there was no graphene in the lower Cu layer to block dislocation propagation. Conversely, most of the gliding dislocations that nucleated in the upper Cu grain, which was 260 nm thick, were effectively blocked by the graphene layer, as evidenced by the fact that the plastic deformation was mostly confined to the upper layer. Because the dislocations could not propagate to the next layer due to the graphene, the upper layer was observed to expand laterally, and the pristine graphene layer was preserved. The lateral bulging of the Cu layer is potentially due to the activation of multiple complex slip systems at high levels of stress, but interfacial sliding could have also allowed the piled-up dislocations to escape to the free surfaces. This in situ study is, therefore, a direct observation of graphene acting as an efficient barrier to gliding dislocations and is consistent with the ex situ high-resolution TEM images of the Cu–graphene multilayers. 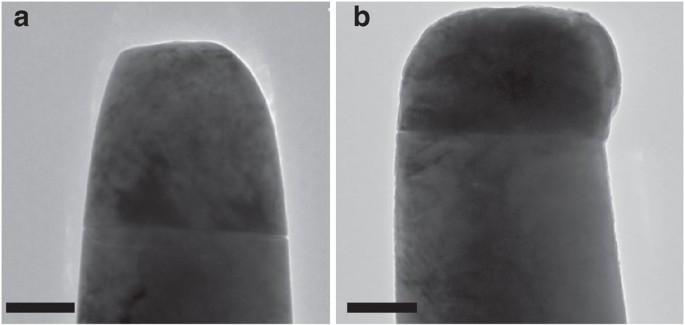Figure 4:In situimaging of the compression of Cu–graphene multilayers. TEM images of a Cu–graphene nanopillar with a single layer of graphene (a) before and (b) after compression testing showing the effectiveness of graphene in blocking gliding dislocations from propagating to the next layer. Scale bar, 100 nm. Figure 4: In situ imaging of the compression of Cu–graphene multilayers. TEM images of a Cu–graphene nanopillar with a single layer of graphene ( a ) before and ( b ) after compression testing showing the effectiveness of graphene in blocking gliding dislocations from propagating to the next layer. Scale bar, 100 nm. Full size image Molecular dynamics simulations An atomistic study of the role of graphene in the composite nanopillars was performed using non-equilibrium molecular dynamics simulations on a model system of 10-nm-diameter Ni nanopillars with a out-of-plane orientation in the presence and absence of a single-layer graphene. To check the validity of the modified embedded atom method (MEAM) potential used, we calculated the stacking fault energy of Ni. The calculated (124 mJ m −2 ) and experimental (125–128 mJ m −2 ) [27] stacking fault energies agreed, justifying the use of MEAM for the present study. To accurately describe the Ni–C interfacial interactions for the case of the graphene-inserted model, the van der Waals type potential was used and optimized to reproduce the ab initio results (see Supplementary Fig. S4 ). The schematic view of the dislocation slip system used in our simulations is summarized in Fig. 5a . In both cases (with and without graphene), we introduced a single pure edge dislocation with gliding on the close-packed slip plane. After equilibration, the initial dislocation line introduced along the direction rotates to to minimize the dislocation line length before spontaneously dissociating into two Shockley partial dislocations of lower energies defined as and . 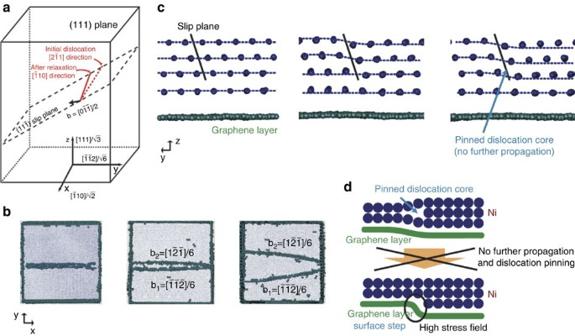Figure 5: MD simulations for single dislocation dynamics. (a) A schematic view of the dislocation slip and model pillar system used in our simulations. (b) Top view of a Ni–graphene nanopillar as a function of compression, where the two Shockley partials are travelling within the slip plane. (c) Side views before the dislocation core arrives (left panel), right after the dislocation core arrives (middle panel), and after the dislocation is pinned and further propagation is blocked at the Ni–graphene interface (right panel). The surface step is not created. Blue-coloured atoms are Ni, and green-coloured atoms are graphene. Blue dotted lines are to guide the reader’s eyes. (d) Schematic figure illustrating the blocking of dislocation propagation at the Ni–graphene interface. Formation of a surface edge structure at the bottom of the upper Ni nanopillar is not favoured due to the high bending stiffness of the graphene. Figure 5: MD simulations for single dislocation dynamics. ( a ) A schematic view of the dislocation slip and model pillar system used in our simulations. ( b ) Top view of a Ni–graphene nanopillar as a function of compression, where the two Shockley partials are travelling within the slip plane. ( c ) Side views before the dislocation core arrives (left panel), right after the dislocation core arrives (middle panel), and after the dislocation is pinned and further propagation is blocked at the Ni–graphene interface (right panel). The surface step is not created. Blue-coloured atoms are Ni, and green-coloured atoms are graphene. Blue dotted lines are to guide the reader’s eyes. ( d ) Schematic figure illustrating the blocking of dislocation propagation at the Ni–graphene interface. Formation of a surface edge structure at the bottom of the upper Ni nanopillar is not favoured due to the high bending stiffness of the graphene. Full size image As the compression load is applied at a fixed displacement rate, the two partial dislocations glide on the plane. The leading partial dislocation moving towards the graphene is eventually pinned near the interface but never penetrates beyond the single layer of graphene due to the strong C–C bond network of the graphene. This observation is consistent with the pile-up of dislocations at the graphene interface observed in the ex situ ( Fig. 2c ) and in situ TEM analyses ( Fig. 4 ). Interestingly, however, the dislocation pinning occurred at the Ni-layer second nearest (or subsurface) to the graphene but did not create a slip step at the interface. More atomistic details of dislocation pinning process are shown in Fig. 5c and are described below. Initially, all Ni atoms are more or less at the perfect lattice sites, and the interfacial Ni atoms have significant attraction (0.20 eV nm −2 from ab initio calculations) to the graphene sheet ( Fig. 5c , left panel). With loading and the arrival of the dislocation core near the interface, subsurface Ni atoms are displaced to accommodate the dislocation core, creating the stress field ( Fig. 5c , middle and right panels). However, the surface Ni atoms interacting directly with the graphene roughly maintain their atomic positions without creating a surface step. The latter observation can be explained by considering the very high bending stiffness of the graphene sheet (bending modulus of 0.192 nN-nm) [28] , as well as the relatively strong Ni/graphene interaction energy (24 eV assuming an experimental pillar size with 200 nm diameter). That is, to create a step step, as shown in the bottom cartoon of Fig. 5d , the graphene sheet must either yield a wrinkled structure on the angstrom length scale to maximize the Ni–graphene interaction, at the expense of the enormous stress fields in the graphene, or sacrifice the substantial total Ni/graphene interaction energy. Both of these events are quite unlikely due to considerable energetic penalty, and thus the dislocation core stays at the subsurface Ni layer ( Fig. 5d upper cartoon). With further loading, defects start to appear throughout the pillar, but no sign of dislocation propagation across the graphene was observed. The nanopillar compression testing of the metal–graphene nanolayered composite revealed that a single atomic layer of graphene can act as an efficient strength enhancer with extremely high strengths corresponding to a reduction in repeat layer spacings. The 100-nm layer spaced Ni–graphene nanolayered composites were determined to have flow stresses at 5% plastic strain up to 52% of the theoretical strength of Ni. Although metal nanolayered composites have previously been reported to show higher strengths by reducing the layer spacing, the strengths of our materials are significantly higher than the reported strengths, with similar metal layer spacings despite the fact that our metal–graphene composite uses only single or double atomic layers of graphene to constrain dislocation motion. For example, the Cu/Ni multilayers with 100-nm Cu and 100-nm Ni repeat layer spacing were reported to have a strength of 0.89 GPa (ref. 4 ), which is only 18.5% and 11.7% of the theoretical strength of Cu and Ni, respectively. Consider a hypothetical Cu/Ni nanolayered composite with a fixed Cu thickness of 100 nm, where the thickness of Ni is systematically reduced from 100 nm to a single atomic layer in thickness; the strengthening effect from this single atomic Ni layer is expected to be significantly lower than our results from the metal–graphene nanolayered composites. Such high strengths of the metal–graphene composites may indicate that the graphene is providing an impermeable interface to dislocations. In addition, an increased degree of strain hardening was observed with a reduction in repeat spacings ( Fig. 3c ), which is indicative of dislocation propagation being effectively blocked at the interface and is therefore consistent with our high-resolution TEM, in situ TEM and MD simulations. The MD simulations indicated that the dislocations are blocked because graphene, which has an extremely high in-plane intrinsic strength and Young’s modulus, cannot be easily perturbed to create a slip step. However, slip step formation is not difficult in metal-only multilayers (for example, Cu/Ni). As a result of the gliding dislocations being blocked by the metal–graphene interface, ultra-high flow stresses were observed for the metal–graphene multilayers. At such high levels of stress, multiple complex slips can be activated, causing lateral bulging of the metal layers, as shown in the TEM ( Figs. 2b and 4b ) and scanning electron microscope ( Fig. 3b ) images of the deformed metal–graphene nanopillars. In addition, the gliding dislocations that are piled up at the metal–graphene interface may escape to the free surface through interfacial sliding to further accommodate the plastic deformation of the metal layers. Therefore, the interfacial shear strength may be an important factor in determining the deformation behaviour of metal–graphene multilayers. Our density functional calculations shown in Supplementary Figure S5 indicate higher interfacial shear strengths for Ni–graphene, which could partially explain the differences in deformation behaviour and strengths of the Cu–graphene versus Ni–graphene multilayers. Our testing methodology used nanopillar compression testing to determine the stress–strain response of the metal–graphene multilayers, but it should be noted that the strengths from our metal–graphene composites are expected to be sustainable without the need for texturing into nanopillars, as the governing length scale of the strength is the repeat layer spacing, not the external dimension of the nanopillar. Therefore, in the results section, the strengths of the metal–graphene layers were compared with the theoretical strengths of the respective metals instead of the strengths of single-crystal nanopillars without graphene, which are known to display external size-dependent strengths [21] , [23] , [24] ; the strengths of pure metal nanopillars increase according to the power–law relationship , where D is the diameter of the nanopillar [21] , [23] , [24] . In attempting to compare the strengths of the metal–graphene nanopillars with those of pure metal nanopillars, it should therefore be recognized that the pure metal nanopillar with a diameter of ~200 nm is already strong due to the small external dimension, but the high strength of the pure metal nanopillar is not sustainable unless the metal is etched into a nanopillar with the same external dimensions. Our metal–graphene multilayers, however, are expected to sustain a high strength without the need to texture into nanopillars because the external dimension of the nanopillar is not the governing length scale. Nevertheless, the Cu–graphene nanopillar compression results were compared with those of pure Cu nanopillars created from six repeated depositions of 100-nm-thick Cu without graphene, as shown in Supplementary Figure S6 , as secondary evidence for the strengthening effect of the graphene. The metal nanopillars etched from a 600-nm-thick Cu thin film on an oxidized Si substrate without graphene had external dimensions similar to the metal–graphene nanopillars (200 nm diameter, 600 nm height) and are shown in Supplementary Figure S6 . The Cu thin film was synthesized using the same procedure as that used for the Cu–graphene multilayers; the 100-nm-thick Cu layer was first deposited on the oxidized Si substrate and then taken out of the sputtering chamber before being reinserted into the sputter system for subsequent layer deposition. This procedure was repeated six times to create a Cu film with a total thickness of 600 nm. The flow stress at 5% plastic strain of the pure Cu nanopillar was 600 MPa, agreeing with the literature value of 5% flow stress for a (111) single-crystal Cu with a 256 nm diameter reported as 580 MPa by Jennings et al . [29] In comparison, our Cu–graphene multilayers with 100-nm repeat layer spacing had a 5% flow stress of 1.5 GPa, which is 2.5 times that of the pure Cu nanopillar. The 3% flow stress for a 200-nm-diameter (111) single-crystal Ni was reported as 1.2 GPa by Frick et al . [30] , while our Ni–graphene nanopillar with 70-nm repeat layer spacing has a 5% flow stress of 4.0 GPa. A clear enhancement in strength can be seen in our metal–graphene multilayers as compared with the pure metal nanopillars, which are already stronger due to external size effects. In summary, we reported a new nanolayered composite strength enhancer design that utilized the full advantages of graphene, namely its 2D geometry and intrinsically high mechanical strength. We have demonstrated a controlled synthesis of Ni– and Cu–graphene nanolayered composites, and their highest strengths are 4.0 GPa at 100 nm and 1.5 GPa at 70 nm, respectively. The measured strengths are as high as 31–52% of the theoretical strengths of the respective metals due to the effective constraint on dislocation propagation across the metal–graphene interface. The remarkable strengthening of the single atomic layer of graphene in our nanolayered composite was confirmed by our ex situ and in situ TEM analyses and MD simulations, which revealed that the high intrinsic mechanical strength of graphene provides an effective barrier against dislocation motion despite the fact that it is only a single atomic layer in thickness. Sample preparation Graphene was grown on a 25-μm-thick Cu foil (Alfa Aesar, Item No. 13382) in a tube furnace by CVD. First, a cut Cu foil was inserted into a quartz tube and then left in vacuum at <10 −4 Torr. The tube was heated to 1,000 °C for 1 h under H 2 (10 sccm). Thereafter, a mixed gas of CH 4 (60 sccm) and H 2 (10 sccm) was injected into the quartz tube for 20 min, and the system was rapidly cooled to room temperature under H 2 flow (10 sccm). Then, the graphene was transferred onto the deposited metal layer to fabricate the metal–graphene multilayer structures. A supporting polymer (PMMA) was spin-coated onto the graphene on the Cu foil to prevent damage to the graphene during transfer. The Cu foil was etched by an aqueous solution (ammonium persulphate), thereby detaching the graphene from the Cu foil. The PMMA with attached graphene was floated in the aqueous solution and cleaned several times with distilled water. The graphene films were transferred by scooping [16] PMMA/graphene films with a metal (Cu or Ni)-deposited substrate. During Ni metal layer depositions, a deposition rate of 1.3 Å s −1 under an e-beam evaporator pressure of 2.5 × 10 −6 Torr was used, and for the Cu layers, a deposition rate of 1.2 Å s −1 under a thermal evaporator pressure of 7.8 × 10 −6 Torr was used. Each substrate was heated to 80 °C for 5 min and then cleaned with acetone for 5 min to remove the PMMA. This process was repeatedly performed to fabricate the repeated layers of graphene and metal. Characterization and nanopillar compression testing A Quanta 3D FEG FIB was utilized to fabricate nanopillars with diameters of 200 nm and heights from 400 to 600 nm. The nanopillar compression testing [21] was performed using a Hysitron TI 750 Ubi nanoindentation system fitted with a flat punch tip at a nominal constant displacement rate of 0.8–1.2 nm s −1 , which translates to an engineering strain rate of 0.002 s −1 . The resulting true stress versus true strain plots were calculated using a constant-volume, homogeneous deformation model [23] . In situ TEM compression tests were performed on a Cu (260 nm)–graphene–Cu (960 nm) nanopillar on Si with a diameter of 205 nm using a Hysitron Picoindenter (PI-95) in a FEI Tecnai G2 F20 TEM. The nanopillars were compressed under in situ TEM at a nominal constant strain rate of 0.002 s −1 . AHVEM, JEM-ARM1300S operated at 1.25 MV, was utilized for detailed TEM analysis to examine the metal–graphene interface. Supplementary Figure S3 shows the TEM image of a Cu–graphene nanopillar with 125-nm repeat layer spacing; the presence of the graphene layer is bound by single grains of Cu in the upper and lower layers. To obtain quantitative grain size measurements, an FEI Tecnai-30 at 200 kV was used to obtain cross-sectional images of Cu–graphene nanolayered composites with 200, 125 and 70-nm repeated layer spacings. As shown in Supplementary Figure S2 , the Cu nanolayers were polycrystalline in nature, and the average grain sizes were 193.6, 143.2 and 158.4 nm for the three different repeated layer spacings of 200, 125 and 70 nm, respectively. Given that the grain sizes of the metal layers were similar to the diameter of the pillar, mostly single-grain metal layers were expected for each nanopillar, thus controlling for the size-dependent plasticity that arises due to the difference in grain sizes. Our nanolayered composite system is well-suited for studying the effect of graphene on blocking dislocation propagation in the absence of any grain boundary sliding effects. Simulation Constant temperature and pressure molecular dynamics (NPT) simulations were performed using LAMMPS [31] . The initial dimension of the simulation box was 11.9472 × 12.708 × 21.9485, nm 3 with 2,89,199 atoms in an FCC–Ni slab configuration. The simulation box was replicated periodically in the z-dimension. The Nosé–Hoover thermostat and barostat with time constants of 0.1 and 1.0 ps, respectively, were used. The MEAM potentials [32] were used to compute pairwise interactions of Ni–Ni and C–C. To describe the Ni–C interfacial interactions, we used the 12-6 Lennard–Jones type of van der Waal’s interaction, where the well depth and equilibrium distance parameters were optimized to reproduce the quantum mechanical interaction energy curve from the dispersion corrected density functional theory calculations [33] ( Supplementary Fig. S5 ). The ab initio equilibrium Ni/graphene distance ( Supplementary Fig. S7 ) suggested that the Ni/graphene interfacial interaction is indeed vdW type, rather than a chemical bonding interaction. The NPT dynamics for this slab were run for 5 ns for equilibration with a 1-fs time step. The initial configurations of a Ni nanopillar and a graphene-inserted nanopillar with a diameter of 9.848 nm were then obtained from this equilibrated FCC–Ni slab system after introducing a dislocation line. For loading experiments, the nanopillars were aligned along the z-direction and non-equilibrium molecular dynamics simulations were performed at a constant displacement rate, where the length of the simulation box along the z-direction decreased at a rate of 0.05 Å ps −1 . For the graphene-inserted Ni pillar, both flexible and rigid graphene models were used for comparison. All simulations were performed at 298 K. How to cite this article: Kim, Y. et al . Strengthening effect of single-atomic-layer graphene in metal–graphene nanolayered composites. Nat. Commun. 4:2114 doi: 10.1038/ncomms3114 (2013).